Ultrasmall copper-based nanoparticles for reactive oxygen species scavenging and alleviation of inflammation related diseases Oxidative stress is associated with many acute and chronic inflammatory diseases, yet limited treatment is currently available clinically. The development of enzyme-mimicking nanomaterials (nanozymes) with good reactive oxygen species (ROS) scavenging ability and biocompatibility is a promising way for the treatment of ROS-related inflammation. Herein we report a simple and efficient one-step development of ultrasmall Cu 5.4 O nanoparticles (Cu 5.4 O USNPs) with multiple enzyme-mimicking and broad-spectrum ROS scavenging ability for the treatment of ROS-related diseases. Cu 5.4 O USNPs simultaneously possessing catalase-, superoxide dismutase-, and glutathione peroxidase-mimicking enzyme properties exhibit cytoprotective effects against ROS-mediated damage at extremely low dosage and significantly improve treatment outcomes in acute kidney injury, acute liver injury and wound healing. Meanwhile, the ultrasmall size of Cu 5.4 O USNPs enables rapid renal clearance of the nanomaterial, guaranteeing the biocompatibility. The protective effect and good biocompatibility of Cu 5.4 O USNPs will facilitate clinical treatment of ROS-related diseases and enable the development of next-generation nanozymes. Inflammation is a natural defensive response to stimulating factors such as infection, injury, and toxins [1] , [2] . However, excessive and uncontrolled inflammation has been demonstrated to cause numerous diseases, such as cardiovascular disease, hepatitis, nephritis, and delayed wound healing [3] , [4] . It has been widely acknowledged that inflammation is intimately associated with oxidative stress [5] , [6] . Reactive oxygen species (ROS) in excessive inflammatory response could aggravate localized tissue injury and lead to chronic inflammation [7] , [8] . Consequently, scavenging ROS with broad-spectrum antioxidants such as N -acetyl cysteine and acetyl- l -carnitine has been regarded as a feasible strategy for the treatment of various inflammatory diseases such as acute liver injury, liver fibrosis, acute or chronic wounds, acute kidney injury (AKI) [9] , [10] . However, poor bioavailability, low stability and efficacy of these drugs limit their clinical application in the treatment of ROS-related diseases [11] , [12] . Advances in nanomedicine have enabled new ways of ROS clearance and thus treatment of ROS-related diseases using various functional nanomaterials [13] , such as carbon [14] , ceria [15] , platinum [16] , redox polymer [17] , and polyphenol nanoparticles (NPs) [18] . Among them, one promising strategy is to develop nanozymes to maintain natural redox balance in biological system, including catalase (CAT), superoxide dismutase (SOD), and glutathione peroxidase (GPx) [19] . Such nanozymes shall have high ROS scavenging ability comparable to native enzymes, broad-spectrum ROS scavenging activities against various toxic ROS species, high stability in harsh disease environment, and rapid clearance from the body to guarantee excellent biocompatibility. Therefore we believe nanomaterials with ultrasmall size (hydrodynamic diameter <5.5 nm) shall be designed because this kind of nanomaterials will have high catalytic activity due to the relatively large surface to volume ratios [20] and rapid renal clearance because they can pass through the glomerular capillary wall in kidney [21] , [22] . Some ultrasmall ROS scavenging nanomaterials have been developed recently. For example, Cai and co-workers reported the synthesis of ultrasmall melanin-based [23] , molybdenum-based [10] , and DNA origami-based [24] antioxidative NPs with preferential renal uptake for AKI treatment. Besides, Qu and co-workers [25] synthesized Cu-TCPP MOF nanodots with SOD mimic property. However, the relatively low catalytic activity and/or high cost of these nanomaterials could impair their clinical translation. It remains a challenge to develop a nanomaterial with simple structure and excellent ROS scavenging ability to enable potential large-scale production and subsequently clinical applications. Copper (Cu), an essential trace element in humans, plays an important role in many enzymes, such as tyrosinase and Cu–Zn SOD [26] , [27] . Therefore, it is reasonable to infer that copper-based nanomaterials can be used to scavenge ROS. For example, Cu NPs have excellent catalytic activity to scavenge H 2 O 2 and O 2 − due to their strong quantum confinement of electrons in the ultrasmall size regime [26] , but cannot eliminate OH· simultaneously [27] . Cuprous oxide (Cu 2 O) NPs possess good catalytic activity and can promote electron transfer reactions to inactivate H 2 O 2 or OH·, thereby partially mimicking peroxidase [13] , [28] . Therefore, we presume that broader-spectrum enzymatic catalytic properties and antioxidant activities could be concurrently achieved by combining Cu 2 O and Cu nanocrystals. Besides, the stability of Cu 2 O coating on Cu NPs can be largely enhanced owing to the effective electron–hole separation between Cu 2 O and Cu, which is also of benefit to improve the overall ROS scavenging ability [29] , [30] . Herein, we report a strategy to synthesize ultrasmall Cu 5.4 O NPs (Cu 5.4 O USNPs) with excellent biocompatibility, enzymatic ROS scavenging abilities, and high renal clearance properties, in order to tackle broad ROS-related diseases (Fig. 1 ). Cu 5.4 O USNPs exhibit remarkable antioxidant efficiency, with a working concentration of approximately 25 ng mL −1 in vitro and 2 μg kg −1 for AKI in vivo. This dosage is at least two orders magnitude lower than all the other reported nanomaterials to treat ROS-related diseases. Furthermore, they possess broad-spectrum ROS scavenging activities and function as CAT, GPx, and SOD analogs. Moreover, the ultrasmall NPs show high renal clearance and achieve an outstanding therapeutic effect against broad ROS-related diseases without any noticeable toxicity. This study provides an attractive strategy to develop ultrasmall copper-based nanozyme systems, which may serve as a blueprint for next-generation nanomedicines used in ROS-related diseases treatment and prevention. Fig. 1: Schematic illustration of Cu 5.4 O ultrasmall nanoparticles in the treatment of ROS-related diseases. Cu 5.4 O ultrasmall nanoparticles with multiple enzyme-mimicking and broad-spectrum ROS scavenging ability are synthesized by a simple and green method. Due to the robust ROS scavenging ability in vivo, Cu 5.4 O ultrasmall nanoparticles exhibit therapeutic effect against broad ROS-related diseases, including acute kidney injury, acute liver injury and diabetic wound healing. Full size image Synthesis and characterization of Cu 5.4 O USNPs USNPs were synthesized by a green, rapid, and cost-effective method (Fig. 2a ). The ratio of Cu 2+ to l -ascorbic acid (AA), reaction temperature, and time were tuned to determine their impact on the particle size and catalytic activity of obtained NPs (Supplementary Figs. 1 – 3 ). A relatively long reaction time is required for obtaining uniform USNPs due to Ostwald ripening (Supplementary Fig. 2 ). Too low and too high temperatures are not feasible to control the reaction (Supplementary Fig. 3 ). The catalytic activity of the obtained copper-based USNPs was almost the same with the feeding ratio of Cu 2+ to AA in the range of 1:10 to 1:40. Therefore, the molar ratio of Cu 2+ to AA was fixed at 1:10 for the following studies. Fig. 2: Preparation and characterization of Cu 5.4 O USNPs. a Schematic preparation of Cu 5.4 O USNPs. b TEM image of Cu 5.4 O USNPs. Inset is the statistical chart of particle size distribution. The cross-sectional area of each particle was measured by using ImageJ Software from the TEM images, with at least 500 particles counted per sample. c Hydrodynamic diameter distribution of the Cu 5.4 O USNPs. d X-ray diffraction (XRD) pattern of the Cu 5.4 O USNPs, the rhombus, and star symbols represent the characteristic peaks of Cu 2 O and Cu, respectively. e XAES spectra of the Cu 5.4 O USNPs. Source data are provided as a Source Data file. Full size image Transmission electron microscopy (TEM) images showed that these Cu 5.4 O USNPs were uniform, with an average diameter of 3.5–4.0 nm in the dry state (Fig. 2b ). The average hydrodynamic diameter of Cu 5.4 O USNPs was approximately 4.5 nm (Fig. 2c ), which meets the kidney filtration threshold of 5.5 nm [21] , [22] , enabling renal uptake, accumulation, and clearance. There were slight increases in the hydrophilic diameters of Cu 5.4 O USNPs in FBS and rat serum (Supplementary Fig. 4a ), possibly due to surface protein adsorption [31] . Cu 5.4 O USNPs were uniformly dispersed, with nearly identical morphologies and particle sizes, indicating that the Cu 5.4 O USNPs were stable in the media for at least 20 days (Supplementary Fig. 4b ). The oxidation state of Cu was investigated through powder X-ray diffraction (Fig. 2d ). The dominant peaks at 2 θ = 41.6°, 50.7°, and 77.5°, which can be assigned to the (111), (200), and (220) lattice planes of Cu(0), are consistent with the presence of face-centered cubic copper. Three additional minor diffraction peaks at 2 θ = 29.6°, 36.4°, and 60.1° can be assigned to the (111), (200), and (220) lattice planes of cuprous oxide (Cu 2 O), respectively. The results suggest that the reaction did not generate pure copper NPs, but rather a mixture of Cu 0 and Cu + (Cu and Cu 2 O NPs). As shown in Fig. 2e , the mass fractions of Cu and Cu 2 O after normalization were calculated based on the peak area of Cu 2p, indicating that the proportions of Cu and Cu 2 O were approximately 3.4. Therefore, the resulting ultrasmall copper-based NPs are denoted as Cu 5.4 O USNPs. ROS scavenging activities of Cu 5.4 O USNPs Three representative ROS, H 2 O 2 , O 2 − , and ·OH, were selected to investigate the ROS scavenging activities of Cu 5.4 O USNPs. As shown in Fig. 3 , the Cu 5.4 O USNPs exhibited a high ROS scavenging activity in a concentration-dependent manner. Approximately 80% of the total H 2 O 2 was decomposed by 200 ng mL −1 Cu 5.4 O USNPs (Fig. 3a ). Approximately half of the O 2 · − was decomposed when treated with 150 ng mL −1 Cu 5.4 O USNPs (Fig. 3b ). More than 80% of the ·OH was scavenged when the Cu 5.4 O USNP concentration was 150 ng mL −1 (Fig. 3c , Supplementary Fig. 5 ). To further confirm the antioxidative properties of Cu 5.4 O USNPs, a free radical scavenging experiment was performed using the classic 2,2′-azino-bis(3-ethylbenzothiazoline 6-sulfonate) (ABTS) radical assay. As presented in Fig. 3d , more than 89% of the free radicals were eliminated by a very low concentration of Cu 5.4 O USNPs (150 ng mL −1 ). Fig. 3: ROS scavenging and multienzyme-like antioxidative activity of Cu 5.4 O USNPs. a H 2 O 2 , b O 2 − , c OH·, and d free radical scavenging ability of Cu 5.4 O USNPs. e H 2 O 2 -scavenging capacities of Cu 5.4 O USNPs and Cu 5.4 O@PEG USNPs. f CAT-like, g SOD-like, and h GPx-like activity of Cu 5.4 O USNPs. i , j The CAT-like activity of the Cu 5.4 O USNPs after different treatments. H 2 O 2 (2 mM) elimination efficiencies of Cu 5.4 O USNPs (250 ng mL −1 ) and natural CAT (40 U mL −1 ), respectively, pretreated with different i temperature and j pH conditions. k Stability test of Cu 5.4 O USNPs (250 ng mL −1 ) when used as CAT-like catalyst at different cycles. The concentration of H 2 O 2 is 2 mM. l XPS analysis of Cu 5.4 O USNPs before and after treatment with H 2 O 2 . In a – j , data represent means ± s.d. from five ( a – d ) or three (e – j ) independent replicates. Source data are provided as a Source Data file. Full size image Compared with the working concentrations of reported metal-based nano-antioxidants for ROS scavenging at cellular level, such as Ce [32] , Au [33] , TiO 2 (ref. [34] ), MnO 2 (ref. [35] ), Co 3 O 4 (ref. [36] ), and V 2 O 5 (ref. [37] ), which are typically in the range of 20–50 μg mL −1 in vitro, the working concentration of Cu 5.4 O USNPs (25 ng mL −1 ) was 2–3 orders of magnitude lower, indicating higher antioxidant efficacy. The working concentration of Cu 5.4 O USNPs was 200-fold lower than that of previously reported Cu x O ( x = 1−2) [19] for the same H 2 O 2 -scavenging capacity. Approximately 80–90% of H 2 O 2 (1 mM) can be scavenged by 0.4 mg mL −1 of vitamin C [38] , whereas 200 ng mL −1 of Cu 5.4 O USNPs could scavenge approximately 85% of H 2 O 2 (2 mM). 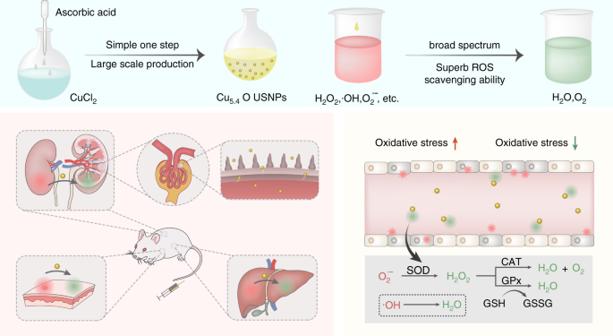Fig. 1: Schematic illustration of Cu5.4O ultrasmall nanoparticles in the treatment of ROS-related diseases. Cu5.4O ultrasmall nanoparticles with multiple enzyme-mimicking and broad-spectrum ROS scavenging ability are synthesized by a simple and green method. Due to the robust ROS scavenging ability in vivo, Cu5.4O ultrasmall nanoparticles exhibit therapeutic effect against broad ROS-related diseases, including acute kidney injury, acute liver injury and diabetic wound healing. Therefore, Cu 5.4 O USNPs showed much stronger H 2 O 2 -scavenging efficiency (approximately 2000-fold) than commonly used small molecular antioxidants, such as vitamin C. To the best of our knowledge, the working concentration of Cu 5.4 O USNPs was also the lowest among all ROS scavenging nanomaterials that have been reported so far (Supplementary Table 1 ). Mechanism of ROS scavenging activities of Cu 5.4 O USNPs Since AA has strong antioxidant activity and can eliminate harmful free radicals both in vitro and in vivo [39] , we initially suspected that the ROS scavenging activities of Cu 5.4 O USNPs originated from the surface-coated AA. We used chemically inert HS-PEG-OH to replace AA molecules on the surface of Cu 5.4 O USNPs (Supplementary Fig. 6 ). Surprisingly, the H 2 O 2 -scavenging abilities of Cu 5.4 O and Cu 5.4 O@PEG USNPs were very similar (Fig. 3e ), suggesting that the presence of AA is not essential for the excellent ROS scavenging abilities of Cu 5.4 O USNPs. According to the previous reports [40] , [41] and our results in Supplementary Figs. 7 and 8 , the AA molecules were possibly converted into dehydroascorbic acid through oxidation of Cu 2+ , and thus lost their reduction activity. Multienzyme-like antioxidative activity of Cu 5.4 O USNPs We further investigated the antioxidant enzyme-mimetic activities of Cu 5.4 O USNPs. Among biologically relevant ROS, H 2 O 2 is of greatest importance because of its membrane permeability, longer half-life than O 2 − and ·OH, and consequently highest intracellular concentration [42] . Therefore, we focused on the CAT-like property of Cu 5.4 O USNPs, which was responsible for decomposition of H 2 O 2 . As shown in Fig. 3f , the concentration-dependent CAT-like activity of Cu 5.4 O USNPs was investigated. Terephthalic acid (TPA) was used as a fluorescence probe, which reacts with ·OH from H 2 O 2 , forming highly fluorescent 2-hydroxyterephthalic acid. Gradual reduction of fluorescence intensity was observed as the concentration of Cu 5.4 O USNPs increased (Supplementary Fig. 9 ). Gradual reduction in the characteristic absorbance of H 2 O 2 at 240 nm (Supplementary Fig. 10a ) and gradual enhancement of the O 2 content (Supplementary Fig. 10b ) were observed with a prolonged reaction time in the presence of Cu 5.4 O USNPs. A steady-state kinetic assay was performed to confirm the enzymatic activity by varying the concentration of H 2 O 2 in the presence of Cu 5.4 O USNPs. This reaction showed typical Michaelis–Menten kinetics (Supplementary Fig. 11 ). The K m value of the Cu 5.4 O USNPs with H 2 O 2 as the substrate was 0.065 mM, and the V max value was 3.92 × 10 −6 Ms −1 . The K m value of Cu 5.4 O USNPs was smaller than that of natural CAT (0.134 mM), indicating that our Cu 5.4 O USNPs possessed greater affinity for substrate H 2 O 2 , possibly due to their ultrasmall size and greater numbers of exposed active sites. Moreover, the concentration-dependent SOD-like activity of Cu 5.4 O USNPs was also investigated. As shown in Fig. 3g , the percentage of formed formazan reduced significantly in the presence of Cu 5.4 O USNPs, indicating the SOD-like activity of Cu 5.4 O USNPs. According to the previous literature, the EC 50 (an indicator for comparing the efficiencies of enzymes and enzyme mimics) of native Cu–Zn SOD [25] , [43] was 41.6 ng mL −1 . The EC 50 of Cu 5.4 O USNPs was calculated to be 191.4 ng mL −1 . Thus, the EC 50 of Cu 5.4 O USNPs was approaching 21.7% of the native SOD activity, which was nearly twice as much as that of the Cu-TCPP MOF nanodots (12.6% of native SOD activity) reported by Qu and co-workers [25] . Besides, the SOD-like activity of Cu 5.4 O USNPs was further confirmed by electron paramagnetic resonance (EPR) spectroscopy (Supplementary Fig. 12 ). In addition, Cu 5.4 O USNPs also displayed concentration-dependent GPx-like activity, eliminating H 2 O 2 and catalyzing the oxidation of reduced glutathione (Fig. 3h ). Natural enzymes often exhibit intrinsic shortcomings, such as low operational stability, temperature and pH sensitivity, and recycling difficulties. Hence, the thermal and pH stabilities of Cu 5.4 O USNPs were investigated and compared with those of the natural enzyme CAT. The results (Fig. 3i, j ) suggested that the stabilities of Cu 5.4 O USNPs when exposed to pH and temperature variations were significantly greater than those of natural CAT. Besides, the recycled Cu 5.4 O USNPs showed nearly identical catalytic activity as the original solution (Fig. 3k ), indicating good stability and recyclability of Cu 5.4 O USNPs. The X-ray photoelectron spectroscopy (XPS) spectra of the Cu 2 p core level region for Cu 5.4 O and Cu 5.4 O oxidized by H 2 O 2 showed only two intense peaks at 932.4 and 952.0 eV for Cu 5.4 O USNPs before and after oxidation, which were assigned to the binding energies of Cu 2 p 3/2 and Cu 2 p 1/2 ; these corresponded to Cu + and/or Cu 0 species, respectively (Fig. 3l ). Upon interaction with H 2 O 2 , the positions of the two main peaks did not shift and new peaks rarely appeared. Hence, we concluded that the ROS scavenging performance of Cu 5.4 O USNPs can be attributed to its intrinsic multienzyme-mimicking properties. Scavenging ROS ability in vitro Compared with the glomerulus, renal tubules are more susceptible to oxidative stress in AKI [44] . Therefore, protection of renal tubules against ROS damage and subsequent initiation of a cascade of pathological processes during the early stage of AKI would significantly reduce kidney dysfunction [44] . For this analysis, the human embryonic kidney 293 (HEK293) cell line was used to examine the cytoprotective properties of Cu 5.4 O USNPs against ROS damage in vitro. As shown in Fig. 4a , the intracellular ROS level (green fluorescent signal) of HEK293 cells increased dramatically after treatment with 250 μM H 2 O 2 , leading to abnormal and shrunken cell morphology. In comparison, the intracellular ROS level obviously decreased when the cells were pretreated with Cu 5.4 O USNPs. Quantitative analysis of intracellular ROS levels via flow cytometry further confirmed this trend (Fig. 4b, c , Supplementary Fig. 13a ). The results of CCK-8 analysis (Fig. 4d ) revealed that an extremely low concentration (25 ng mL −1 ) of Cu 5.4 O USNPs was able to completely protect the cells against 250 μM H 2 O 2 , which is higher than the concentration in the classical AKI pathological microenvironment. Fig. 4: Scavenging ROS with Cu 5.4 O USNPs in vitro. a Representative ROS staining (green fluorescence) of HEK293 cells under different treatment conditions. b ROS levels in untreated and Cu 5.4 O USNPs-treated HEK293 cells incubated with 250 μM H 2 O 2 . c Statistical analysis of ROS levels in HEK293 cells under different treatment conditions. d In vitro cell viabilities of HEK293 cells under different treatment conditions. e FACS results of cell apoptosis and necrosis distribution in untreated and Cu 5.4 O USNPs-treated HEK293 cells. f Statistical analysis of necrotic and apoptotic cell ratios in HEK293 cells under different treatment conditions. In c , d and f , data represent means ± s.d. from four ( c , f ) or six ( d ) independent replicates. *** P < 0.001; n.s., no significance, one-way ANOVA. Source data are provided as a Source Data file. Full size image We further examined the effect of Cu 5.4 O USNPs against H 2 O 2 -induced cell apoptosis and necrosis via flow cytometry. In Fig. 4e, f and Supplementary Fig. 13b , the addition of Cu 5.4 O USNPs significantly reduced the ratios of apoptotic and necrotic cells induced by H 2 O 2 treatment, further confirming the ROS scavenging and cytoprotective properties of Cu 5.4 O USNPs at the cellular level. As shown in Supplementary Fig. 14 , Cu 5.4 O USNPs could be found in the mitochondria of cells, which was consistent with previous reports that ultrasmall NPs could easily enter the mitochondria through the mitochondrial permeability transition pore [45] , [46] , indicating that Cu 5.4 O USNPs could alleviate mitochondrial oxidative stress and maintain mitochondrial function. Besides, Cu 5.4 O USNPs could also be observed in the phagosome, suggesting that Cu 5.4 O USNPs might enter into the cells through phagocytosis. In vitro and in vivo biocompatibility of Cu 5.4 O USNPs The CCK-8 assay results (Supplementary Fig. 15 ) suggested that Cu 5.4 O USNPs at test concentrations did not exhibit noticeable cytotoxicity. HEK293 cells exposed to 200 ng mL −1 Cu 5.4 O USNPs for 48 h showed normal polygonal cytoskeleton morphology (Supplementary Fig. 16 ), indicating good biocompatibility. Such results are in accordance with previously findings that copper NPs are generally non-toxic at relatively low concentrations (<5 μg mL −1 ) [47] . Additionally, hemolysis rate of nanomaterials must be less than 5% to ensure safety during intravenous administration [48] , [49] . As shown in Supplementary Fig. 17 , the hemolysis rate of 500 ng mL −1 Cu 5.4 O USNPs, which is 10-fold greater than the concentration applied in vivo to treat AKI (2 μg kg −1 , corresponding to 50 ng mL −1 for a 25 g mouse with 1 mL of blood), was less than 5%. Next, we evaluated the impacts of Cu 5.4 O USNPs (4 μg kg −1 , twofold greater than the concentration used to treat AKI) on blood chemistry, inflammatory cytokine levels, and major organ histopathology in healthy mice to reveal their in vivo biocompatibility. As shown in Fig. 5a and Supplementary Fig. 18 , no necrosis, congestion, or hemorrhage was observed in the heart, liver, spleen, and lung at 1 and 30 days after single dose intravenous injection of Cu 5.4 O USNPs. Moreover, no distinguishable inflammatory lesions or tissue damage were observed in the glomerulus, tubules, collecting ducts, and urethra at 24 h after single dose intravenous injection of Cu 5.4 O USNPs (Fig. 5b ). Fig. 5: In vivo biocompatibility assessment of Cu 5.4 O USNPs. a Evaluation of in vivo toxicity of Cu 5.4 O USNPs to major organs (heart, liver, spleen, and lung) at 24 h after intravenous administration. b Assessment of in vivo toxicity of Cu 5.4 O USNPs to the kidney at 24 h after intravenous administration. c Serum levels of inflammatory factors of interleukin-6 (IL-6) and tumor necrosis factor alpha (TNF-α). d Serum levels of liver function indicators: aspartate transaminase (AST) and alanine transaminase (ALT). e Serum levels of kidney function indicators: blood urea nitrogen (BUN) and creatinine (CRE). f – j Blood parameters in normal mice (control group), and mice intravenously injected with Cu 5.4 O USNPs, 24 h after injection. In c – j , data represent means ± s.d. from five independent replicates. Source data are provided as a Source Data file. Full size image As shown in Fig. 5c , the serum levels of interleukin-6 (IL-6) and tumor necrosis factor-α (TNF-α) in the Cu 5.4 O USNPs-treated group were identical to the levels in the control group ( P > 0.05), indicating that Cu 5.4 O USNPs would not trigger obvious immune responses in vivo at the tested concentration. The serum biochemistry analysis results (Fig. 5d, e ) showed that serum concentrations of liver function indicators (aspartate transaminase (AST) and alanine transaminase (ALT)) and kidney function indicators (BUN and CRE) in the Cu 5.4 O USNPs-treated group were similar to those in the control group ( P > 0.05), revealing good biocompatibility in the liver and kidney. Moreover, the results of complete blood panel analysis (Fig. 5f–j ) showed no obvious differences in the hematology of the Cu 5.4 O USNPs-treated group when compared to that of the control group ( P > 0.05). We also investigated the accumulation of Cu 5.4 O USNPs in the major organs after repeated daily administration of Cu 5.4 O USNPs for seven consecutive days. As shown in Supplementary Fig. 19 , the liver and kidneys exhibited higher normalized dosage distribution of Cu 5.4 O USNPs, reaching 7.92 and 7.97 %ID g −1 respectively, while the distributions of NPs in the heart, spleen, lung, and blood reached 2.25, 5.07, 3.02, and 2.84 %ID g −1 , respectively. As shown in Supplementary Fig. 20 , Cu 5.4 O USNPs could be found in the tissues of major organs by TEM, which is consistent with the above results. The in vivo toxicity of Cu 5.4 O USNPs accumulated in the major organs after repeated intravenous administration was also evaluated. As shown in Supplementary Fig. 21 , no necrosis, congestion, or hemorrhage was found in the heart, liver, spleen, lung, and kidney of the mice after intravenous repeated administration. Besides, the serum biochemistry analysis and complete blood panel analysis (Supplementary Fig. 22 ) results further indicated no obvious toxicity of Cu 5.4 O USNPs. All the results confirmed that the synthesized Cu 5.4 O USNPs exhibited negligible short-term and long-term in vivo toxicity. Pharmacokinetics and biodistribution of Cu 5.4 O USNPs in mice The time-dependent blood circulation profiles of Cu 5.4 O USNPs in Fig. 6a demonstrated a classical two-compartment pharmacokinetic model. The terminal elimination half-lives of the central component and peripheral component were 0.77 and 71.2 h, respectively. The biodistribution of Cu 5.4 O USNPs in the major organs of AKI mice at 24 h post injection was detected by inductively coupled plasma-atomic emission spectrometry. As shown in Fig. 6b , the kidney exhibited the highest normalized dosage distribution of Cu 5.4 O USNPs (4.4 %ID g −1 ), while the distributions of NPs in the heart, liver, spleen, and lung reached 0.89, 3.2, 2.1, and 0.94 %ID g −1 , respectively. The accumulation of Cu 5.4 O USNPs in the kidneys might be attributed to the high renal uptake resulting from their ultrasmall hydrodynamic diameter (approximately 4.5 nm) and excellent hydrophilicity. Previous studies showed that the size threshold of the glomerular basement membrane (GBM) was approximately 5.5 nm, and nanomaterials with a diameter less than 5.5 nm could be effectively cleared from the blood to the renal tubules through the GBM [50] , [51] , [52] . As shown in Supplementary Fig. 23 , TEM analysis revealed Cu 5.4 O USNPs in the urine of AKI mice after injection, further confirming that the Cu 5.4 O USNPs could pass through the GBM to the tubules and then undergo excretion in the urine. The time-dependent accumulation of Cu 5.4 O USNPs in the kidneys of normal and AKI mice indicated that Cu 5.4 O USNPs could effectively accumulate in the kidneys, regardless of the permeability of the GBM (Supplementary Fig. 24 ). Moreover, time-dependent accumulation of Cu 5.4 O USNPs in the urine revealed that renal clearance is the main excretion pathway for these particles, rather than intestinal excretion (Fig. 6c ). Approximately 70% of Cu 5.4 O USNPs could be excreted within 48 h post injection (60% through the kidneys and 10% through the intestine), suggesting relatively rapid clearance and potentially low long-term toxicity of Cu 5.4 O USNPs. Fig. 6: Pharmacokinetics, biodistribution, and clearance of Cu 5.4 O USNPs in AKI mice. a In vivo blood pharmacokinetic curves after intravenous injection of Cu 5.4 O USNPs. b Biodistribution of Cu 5.4 O USNPs in major organs at 24 h post injection. c Cumulative urine and feces excretion at different time points. d Biodistribution of Cu 5.4 O USNPs in renal tissues by TEM observation. Red dashed lines indicate the magnified area. Dots with red pseudocolor indicate Cu 5.4 O USNPs. In a – c , data represent means ± s.d. from three independent replicates. Source data are provided as a Source Data file. Full size image To further analyze the distribution of Cu 5.4 O USNPs in the kidneys, renal tissues were collected, ultrathin sectioned, and observed under TEM. As shown in Fig. 6d and Supplementary Fig. 25 , Cu 5.4 O USNPs (arrowheads) were found in the GBM, urinary space, and epithelial cell cilia of renal tubules, confirming that the Cu 5.4 O USNPs could pass through the GBM and reach tubules containing urine. In vivo therapeutic efficacy of Cu 5.4 O USNPs on AKI mice The therapeutic effect of Cu 5.4 O USNPs on AKI mice was tested (Fig. 7a ). As shown in Fig. 7b , compared with the control group (90% of mice died within 5 days following establishment of the AKI model), all AKI mice treated with Cu 5.4 O USNPs survived for more than 14 days. In addition, AKI mice treated with Cu 5.4 O USNPs exhibited a weight increase similar to that of healthy mice (Fig. 7c ), while control AKI mice underwent dramatic body weight loss within 24 h. Furthermore, the serum levels of two important kidney function indicators, BUN and CRE levels, of AKI mice treated with Cu 5.4 O USNPs were significantly lower than those of AKI mice in the control group ( P < 0.001, Fig. 7d, e ). There were no detectable differences in BUN and CRE levels between healthy mice and Cu 5.4 O USNPs-treated AKI mice ( P > 0.05), confirming the excellent therapeutic efficacy of Cu 5.4 O USNPs in the treatment of glycerol-induced AKI. Fig. 7: Ttherapeutic efficiency of Cu 5.4 O USNPs on AKI mice. a Schematic illustration of the establishment and treatment schedule of AKI mice. b Survival curves of AKI mice with different treatment. c Weight variation of AKI mice at 24 h after treatment with Cu 5.4 O USNPs. Serum levels of d CRE and e BUN in AKI mice at 24 h after different treatment. f H&E staining of kidney tissues from each group. Triangles indicate the formation of casts. g Dihydroethidium (red fluorescence) and DAPI (blue fluorescence) staining of kidney tissues from each group. h SOD, i KIM-1, and j HO-1 levels measured in renal tissue homogenates from each group. In c – e and h – j , data represent means ± s.d. from four independent replicates (*** P < 0.001; n.s., no significance, One-way ANOVA). Source data are provided as a Source Data file. Full size image In kidney diseases, the precipitation of denatured proteins in tubules forms a cast structure, which is regarded as an important diagnostic marker of pathological changes. As shown in Fig. 7f , many casts (marked as triangles) could be found in the renal tissues of AKI mice, whereas only a few casts could be observed in AKI mice that were treated with Cu 5.4 O USNPs, suggesting that renal tissue integrity was maintained via adoption of the NPs. To further demonstrate the therapeutic activity of Cu 5.4 O USNPs acting as a ROS scavenger in vivo, NAC molecules with different concentrations (8, 40, and 160 mg kg −1 ) were intravenously injected into AKI mice as controls. As shown in Supplementary Fig. 26 , the CRE, BUN levels and survival percentage of AKI mice treated with Cu 5.4 O USNPs (at 2 μg kg −1 concentration) were similar to those of AKI mice treated with 160 mg kg −1 of NAC, which was also in accordance with the histological analysis of renal tissues. The overall results indicated the in vivo ROS scavenging activity of Cu 5.4 O USNPs. The ROS levels and SOD activity in the kidneys were further investigated to understand the molecular mechanism underlying the protection process. Compared with PBS-treated AKI mice, the levels of superoxide in Cu 5.4 O USNPs-treated AKI mice were significantly reduced, reaching the levels exhibited in normal mice (Fig. 7g , Supplementary Fig. 27 ). As shown in Fig. 7h , the renal SOD activity in Cu 5.4 O USNPs-treated AKI mice was similar to that of healthy mice, whereas a significant reduction in SOD activity was observed in AKI mice in the control group ( P < 0.001). This result suggested that Cu 5.4 O USNPs could protect renal cells by functioning as antioxidants to scavenge ROS and maintain SOD activity in vivo. Furthermore, the renal expression levels of two important kidney injury biomarkers [53] , [54] , heme oxygenase-1 (HO-1) and kidney injury molecule-1 (KIM-1), were detected. As shown in Fig. 7i, j , compared with AKI mice in the control group, Cu 5.4 O USNPs-treated AKI mice exhibited significantly reduced levels of KIM-1 and HO-1 ( P < 0.001), consistent with the results we found for CRE and BUN. The cisplatin-induced AKI (Cis-AKI) mouse model was also used to demonstrate the broad application of Cu 5.4 O USNPs for ROS-mediated AKI diseases. As shown in Supplementary Fig. 28 , kidney function examination and histological analysis revealed that kidney damage in Cis-AKI mice treated with Cu 5.4 O USNPs was significantly lower than that in Cis-AKI mice treated with PBS ( P < 0.001; P < 0.05), confirming the therapeutic effect of Cu 5.4 O USNPs against Cis-AKI. Therapeutic effect on acute liver injury and wound healing It is intriguing for us to discover whether the Cu 5.4 O USNPs could be applicable to ROS-related pathological conditions other than AKI. Therefore, acetaminophen (APAP)-induced acute liver injury (AILI) and full-thickness skin defect were chosen as the representative ROS-related disease models as well. As shown in Fig. 8a, b , the ALT and AST levels of Cu 5.4 O USNPs-treated AILI mice were significantly lower than those of AILI mice without treatment ( P < 0.001), indicating the excellent therapeutic effect of Cu 5.4 O USNPs on AILI. Histological observation of liver tissues further confirmed the therapeutic effect of Cu 5.4 O USNPs on AILI (Fig. 8c ). Fig. 8: Therapeutic efficiency of Cu 5.4 O USNPs on AILI and wound healing. Serum levels of a AST and b ALT in AILI mice at 24 h after different treatment. c H&E staining of liver tissues from each group. Blue dashed lines indicate the range of hepatic necrosis. The percentage of d closed diabetic wound area and representative macroscopic appearance of e diabetic wound at different time points. A 6-mm-diameter standard green disc was used as the reference when taking photos. f Representative histological images and g quantitative determination of the length of regenerated epidermis on day 15 post-surgery. The yellow double-headed arrows indicate the regenerated epidermis. h Representative histological images and i quantitative measurement of granulation tissue thickness on day 15 post-surgery. The yellow double-headed arrows indicate the granulation tissue. In a , b , data represent means ± s.d. from five independent replicates (one-way ANOVA). In d , g and i , data represent means ± s.d. from three independent replicates (Student’s t -test, ** P < 0.01; *** P < 0.001). Source data are provided as a Source Data file. Full size image Elevated ROS production in the wound site has also been implicated in delaying wound healing [32] , [55] , especially in chronic diabetic wounds where high glucose and proinflammatory environment caused the large production of ROS in the wound bed [56] , [57] . As shown in Fig. 8d, e , the diabetic wound healing rate of Cu 5.4 O USNPs group was always significantly faster than that of the corresponding control group on days 4, 7, 9, and 15 post-surgery ( P < 0.01). The results clearly indicated that Cu 5.4 O USNPs could accelerate the diabetic wound healing process. As shown in Fig. 8f–i , the length of newly regenerated epidermis and the thickness of granulation tissue in the Cu 5.4 O USNPs group were significantly greater than those in the control group, further confirming that Cu 5.4 O USNPs could promote diabetic wound healing. Therapeutic mechanisms of Cu 5.4 O USNPs on AKI To further elucidate the underlining therapeutic mechanisms, AKI was chosen as the representative disease model for further transcriptomics analysis. An unguided principal component analysis (PCA) of the data revealed substantially different transcriptomic profiles between Cu 5.4 O- and PBS-treated AKI mice kidneys (Fig. 9a ). The Venn diagram in Fig. 9b showed that 13025 genes were co-expressed by two groups, while 584 genes were exclusively expressed by Cu 5.4 O-treated group. Volcano plots (Fig. 9c ) showed 5819 significantly differentially expressed genes (DEGs), of which 2813 and 3006 genes were upregulated and downregulated, respectively. Fig. 9: Therapeutic mechanisms of Cu 5.4 O USNPs on AKI. a Principal component analysis (PCA) was performed based on differentially expressed genes from the kidneys of two groups. Each data point corresponds to the PCA analysis of each sample. b Venn diagram of the transcriptomic profiles between Cu 5.4 O USNPs and PBS groups. c Volcano plots showing the identified upregulated and downregulated genes by Cu 5.4 O USNPs. d KEGG pathway enrichment analysis of the identified differentially expressed genes. The 20 most significantly enriched pathways are shown. Heat maps of significantly e upregulated and f downregulated genes involved in the oxidative stress after Cu 5.4 O USNPs treatment (fold change ≥2 and P < 0.05). g Protein–protein interaction network of differentially expressed genes involved in the oxidative stress. h qRT-PCR analysis of the mRNA expression levels of antioxidant genes. i Western blot analysis of the expression of phospho-NF-κB p65, total NF-κB p65, phospho-IκB-α, and total IκB-α in kidney tissues of AKI mice. Serum levels of j TNF-α and k IL-1β. Renal levels of l TNF-α and m IL-1β. In h , j–m , data represent means ± s.d. from three independent replicates, and P values were calculated by Student’s t -test ( h ) and one-way ANOVA ( j–m ). * P < 0.05; ** P < 0.01; *** P < 0.001. Source data are provided as a Source Data file. Full size image Kyoto Encyclopedia of Genes and Genomes (KEGG) pathway enrichment analysis (Fig. 9d ) indicated that the glutathione (GSH) metabolism, MAPK signaling pathway, and TNF signaling pathways were highly associated with the therapeutic mechanisms of Cu 5.4 O USNPs. Literature has reported that ROS could activate the MAPK signaling pathway to induce renal cell apoptosis and the release of local or systemic inflammatory mediators to aggravate renal injury [58] , [59] , [60] . Notably, the MAPK signaling pathway (Supplementary Fig. 29 ) was significantly inhibited after Cu 5.4 O USNPs treatment, indicating that Cu 5.4 O USNPs could alleviate renal injury via inhibiting the MAPK signaling pathway through decreasing the ROS level. In addition, it has been reported that ROS could promote the production of proinflammatory cytokines (e.g. TNF-α, IL-1β, IL-6) [58] , [61] and that TNF-α could further trigger a strong cascade inflammatory response throughout the TNF-α/MAPK and TNF-α/NF-κB signaling pathways, resulting in an excessive inflammation response and more pronounced renal damage [62] . Notably, the TNF signaling pathway (Supplementary Fig. 30 ) was also significantly inhibited after Cu 5.4 O USNP treatment, suggesting that other therapeutic mechanisms of renal protection occur through inhibiting the TNF signaling pathway. We also investigated the impact of Cu 5.4 O USNPs on the expression of genes related to oxidative stress. As shown in Fig. 9e, f , several important antioxidant genes, including SOD1, SOD2, SOD3, GPX1, GPX3, GPX4, GPX6, and CAT , were significantly upregulated after the Cu 5.4 O USNPs treatment. The expression trend of the SOD and HMOX1 genes was consistent with the aforementioned result regarding the SOD (Fig. 7h ) and HO-1 proteins level (Fig. 7j ) in AKI mice, respectively. Moreover, the genes associated with oxidative stress that significantly changed after Cu 5.4 O USNP treatment were used in the protein–protein interactions network analysis (Fig. 9g ). We discovered that the neighboring proteins connected to the leading proteins contained SOD1, SOD3, CAT, etc., indicating that these genes play an important role in ROS scavenging after Cu 5.4 O treatment. As shown in Fig. 9h , the mRNA expression levels of antioxidant genes in Cu 5.4 O-treated mice kidneys were significantly higher than those of the corresponding control group, confirming that Cu 5.4 O USNPs could maintain a high expression of antioxidant genes in AKI by protecting renal cells from ROS damage. The phosphorylation of NF-κB and IκB were significantly enhanced in the AKI mice (Fig. 9i , Supplementary Fig. 31 ), indicating the activation of NF-κB signaling pathway in AKI. Besides, the phosphorylation of NF-κB and IκB were significantly decreased in the Cu 5.4 O USNPs group, indicating that the NF-κB signaling pathway was inhibited after Cu 5.4 O USNPs treatment, which was also in accordance with the aforementioned transcriptomics analysis result (Supplementary Fig. 30 ). We also detected the downstream inflammatory factors of the NF-κB signaling pathway. As shown in Fig. 9j–m , Cu 5.4 O USNPs could significantly reduce the serum and tissue levels of TNF-α and IL-1β, indicating that Cu 5.4 O USNPs could protect kidney tissues from oxidative stress by inhibiting the production of excessive proinflammatory factors. Additionally, we found that several important genes related to tissue repair, including fibroblast growth factor 10 ( FGF10 ), hepatocyte growth factor ( HGF ), NOTCH1, and wingless-type MMTV integration site family member 7A ( WNT7A ), were significantly upregulated after the Cu 5.4 O USNPs treatment (Supplementary Fig. 32a, b ). The protein–protein interaction network further confirmed the importance of these genes in tissue repair and regeneration, as shown in Supplementary Fig. 32c . The overall results indicated in addition to the ROS scavenging ability, Cu 5.4 O USNPs may also promote the expression of genes related to renal repair and regeneration. In summary, we have presented uniform and stable Cu 5.4 O USNPs that mimic an intracellular antioxidant enzyme-based defense system. The distinctive advantages of Cu 5.4 O USNPs are the ultrasmall particle size, rapid renal clearance, high biocompatibility, and broad ROS scavenging abilities. Both in vitro and in vivo experiments demonstrated excellent biocompatibility and cytoprotective effects of Cu 5.4 O USNPs against ROS-mediated damage. Cu 5.4 O USNPs could be applicable to various ROS-related pathological conditions such as AKI, ALI, and diabetic wound. Taken together, the synthesized ultrasmall Cu 5.4 O USNPs with robust ROS scavenging abilities and excellent biocompatibility could represent a promising antioxidant for the treatment of AKI and other oxidative stress-related diseases. We expect that our findings will promote the development of nanomaterials with multiple enzyme-mimicking properties and enable further clinical applications of copper-based ROS scavengers in biomedical treatment and research. Materials Cupric chloride (CuCl 2 ), l -ascorbic acid (AA), and sodium hydroxide (NaOH) were purchased from J&K Scientific (Beijing, China). 3,3′,5,5′-Tetramethylbenzidine (TMB) and 2,2′-azino-bis(3-ethylbenzthiazoline-6-sulfonate) (ABTS) was bought from Macklin (Shanghai, China). Acetic acid (HAc), sodium acetate (NaAc), and potassium persulfate (K 2 S 2 O 8 ) was obtained from Sigma-Aldrich (Shanghai, China). Thiol-polyethylene glycol-OH (SH-PEG-OH) (Mw: 1000 Da) was purchased from Yare Biotech. Inc. (Shanghai, China). Catalase (purified powder from bovine liver), superoxide dismutase (purified powder from bovine erythrocytes), and peroxidase (purified powder from horseradish roots) were from Sangon Biotech (Shanghai, China). Phosphate-buffered saline (PBS, pH 7.4, Na 2 HPO 4 –NaH 2 PO 4 , 10 mM) solution was prepared in the laboratory. All chemicals and reagents were of analytical grade and used as received without further purification. Ultrapure water (18.2 MΩ cm −1 at 25 °C) purified by a Milli-Q system was used throughout the experiment. Instrumentation TEM imaging was conducted on a Tecnai G220 (Shimadzu, Japan) at 200 keV. The sample was prepared by dispersing a small amount of freeze-dried powder in the PBS. Then, the suspension was dropped on 230 mesh copper TEM grids covered with thin amorphous carbon films. Fourier Transform infrared spectroscopy (FTIR) spectra were measured by a FTIR-8300 series spectrometer (Shimadzu, Japan) in the range of 4000–400 cm −1 . The fluorescence spectra were determined by using an F-2500 spectrofluorometer (Hitachi, Japan). The UV-vis spectra were obtained using a Hitachi U-3010 spectrometer (Hitachi, Japan). A dynamic light scattering (DLS) particle size analyzer (Malvern 2000, USA) was used to determine the hydrophilic diameters of the particles. XPS and X-ray Auger electron spectroscopy measurement were performed by an ESCALAB 250 Xi Mg (Thermo Scientific, Japan) X-ray resource. Crystal structure and oxidation state of Cu 5.4 O USNPs were analyzed using X-ray diffractometer (XRD, Bruker AXS D8) with a scan rate of 1 s per step with a step size of 0.02. The concentration of Cu was detected by inductively coupled plasma-atomic emission spectrometry (ICP-AES) (Thermo Scientific, iCAP 7400, USA). The concentration of Cu 5.4 O USNPs used in following studies is calculated based on Cu element. The EPR spectroscopy signal was obtained on a Bruker A300 (X-band) spectrometer (Bruker, Germany). All the measurements were performed at room temperature if not specially mentioned. Synthesis of fluorescent Cu 5.4 O USNPs The Cu 5.4 O USNPs was synthesized according to previous report with some modifications [40] . In a typical preparation process, 10 mM CuCl 2 powders were dissolved in 50 mL deionized water and stirred for 10 min at 80 °C in an oil bath with magnetic stirring. Then, l -ascorbic acid aqueous solution (100 mM, 50 mL) was added slowly to the above CuCl 2 solution. Afterwards, the pH of the solution was adjusted to 8.0–9.0 using NaOH solution (1 M). The mixture was kept at 80 °C for 12 h with constantly stirring. After reaction, the larger aggregates were removed by centrifugation (6577 × g , 15 min), and then the supernatant was dialyzed against water (Mw cutoff: 10,000 Da) for 2 days to remove small molecules. Purified Cu 5.4 O USNPs were concentrated with centrifugation. Surface functionalization of Cu 5.4 O USNPs by SH-PEG-OH In total, 0.1 g Cu 5.4 O USNPs were dispersed into 5 mL water under ultrasonication for 1 min and then stirred for 1 h. In all, 0.1 wt% of SH-PEG-OH was added. The reaction mixture was stirred for another 24 h, dialyzed to remove unreacted SH-PEG-OH molecules, and then concentrated by centrifugal ultrafiltration. H 2 O 2 scavenging activity of Cu 5.4 O USNPs H 2 O 2 scavenging capacity of Cu 5.4 O USNPs was tested by the Hydrogen Peroxide Detection Kit (Nanjing Jiancheng Bioengineering Institute, China). H 2 O 2 reacts with ammonium molybdate to form a stable yellow complex, which displays an absorbance peak at 405 nm. Various concentrations of Cu 5.4 O USNPs (25–200 ng mL −1 ) were incubated with 2 mM H 2 O 2 at 37 °C for 2 h, respectively. After reaction, the concentration of remaining H 2 O 2 was determined according to the manufacturer’s instructions, and the H 2 O 2 -eliminating capacity was calculated. ·OH scavenging activity of Cu 5.4 O USNPs The TMB chromogenic method was performed for ·OH scavenging activity test. The ·OH was generated by the classical Fenton reaction between H 2 O 2 and Fe 2+ , which can convert the TMB to a oxidized TMB (oxTMB) with a characteristic absorption at 652 nm. Therefore, the concentration of remaining ·OH can be determined via monitoring the absorption at 652 nm of oxTMB. In detail, The working test solutions containing 250 μM TMB, 2 mM H 2 O 2 , 1 mM FeSO 4 and different concentrations of Cu 5.4 O USNPs (25–175 ng mL −1 ) in HAc/NaAc buffer (0.5 M, pH 4.5) were prepared in the dark and rest for 5 min. Afterwards, the absorbance peak in 652 nm of the solution was monitored with a UV-vis spectroscopy. The EPR spectroscopy signal was measured by a Bruker A300 spectrometer (Bruker, Germany). Typically, 2 mM H 2 O 2 , 20 μM FeSO 4 , 100 mM DMPO, and different concentration of Cu 5.4 O USNPs (0, 50, 150 ng mL −1 , respectively) were added into the HAc/NaAc buffer (0.5 M, pH 4.5); EPR signal was detected immediately. O 2 − scavenging activity of Cu 5.4 O USNPs The superoxide anion (O 2 − ) scavenging activity was assessed using a superoxide anion assay kit (Nanjing Jiancheng Bioengineering Institute, Nanjing, China) according to the manufacturer’s instructions. Different concentrations of Cu 5.4 O USNPs (0–150 ng mL −1 ) were added to the working solution. The absorbance at 550 nm was measured using a multiple plate reader after standing for 10 min. ABTS radical scavenging activity of Cu 5.4 O USNPs The evaluation of ABTS radical scavenging activity was based on the method reported by Wang et al. [63] . Briefly, the ABTS radicals were generated by reacting 7 mM ABTS stock solution with 2.45 mM potassium persulfate in the dark for 16 h. Then, the ABTS radical solution was diluted by PBS to reach a proper absorbance at 734 nm. Two milliliters Cu 5.4 O USNPs solutions (0, 50, 75, 100, 125, 150 ng mL −1 , respectively) were mixed with 2 mL ABTS solution and placed in dark for 10 min. Then the absorbance peak at 734 nm was monitored with a UV–vis spectroscopy. The ABTS radical scavenging abilities were calculated as follows: 
    ABTS scavenging ratio( %) = ( ( A_control - A_sample)/A_control) × 100,
 (1) where A control is the absorbance of a standard without any radical scavengers, and A sample is the absorbance after the reaction with the radical scavengers, respectively. CAT-like activity of Cu 5.4 O USNPs The CAT-like activity of the Cu 5.4 O USNPs and the steady-state kinetic were assayed using a fluorescence spectroscopy [19] , [36] . Typically, TPA is a non-fluorescent compound, which can react with ·OH, decomposed from H 2 O 2 , to produce a fluorescent aromatic hydroxylated product (2-hydroxyterephthalic acid) with excitation/emission peaks at 315/425 nm respectively. In the presence of CAT or CAT analogs, the H 2 O 2 decomposed into H 2 O and O 2 could not produce the fluorescent 2-hydroxyterephthalic acid. Hence, the CAT-like activity of the Cu 5.4 O USNPs was investigated by monitoring the fluorescence signal of the system. The steady-state kinetic assay of Cu 5.4 O USNPs and CAT were performed to confirm the enzymatic catalysis mechanism, by varying the concentration of H 2 O 2 (0–6 mM) in the presence of Cu 5.4 O USNPs (1000 ng mL −1 ) and H 2 O 2 (0–1 mM) in the presence of CAT. Firstly, 200 μL 1000 ng mL −1 of Cu 5.4 O USNPs solution or 20 U mL −1 CAT was added into the PBS (10 mM, pH 7.4), different concentrations of H 2 O 2 were added and incubated at 40 °C for 5 h. Finally, the TPA in 2 mM NaOH was added and the fluorescence spectra of the resultant solution were recorded under an excitation of 315 nm, and the variation of fluorescence emission at 425 nm was adopted to quantify remaining H 2 O 2 . Apparent kinetic parameters were calculated on the flowing basis of the Michaelis–Menten equation [64] . V_0 = V_max[ S ]/[ S ] + K_m,
 (2) where V 0 is the initial catalytic rate, V max is the maximum rate conversion, which is obtained when the catalytic sites on the enzyme are saturated with substrate concentration, and K m is the apparent Michaelis–Menten equation. Maximum initial velocity ( V max ) and Michaelis–Menten constant ( K m ) were obtained using Lineweaver–Burk plots [65] . SOD-like activity of Cu 5.4 O USNPs The SOD-like activity of Cu 5.4 O USNPs was determined by formazan formation using a SOD assay kit (WST-1 method) (Nanjing Jiancheng Bioengineering Institute, Nanjing, China) [19] . Briefly, O 2 − was generated through the oxidation of xanthine by xanthine oxidase (XO), which can convert the WST-1 into WST-1 formazan with a characteristic absorption at 450 nm. The formazan concentration was determined at 450 nm using a multiple plate reader. The SOD-like activity of Cu 5.4 O USNPs was further confirmed with EPR spectroscopy. Briefly, a series of samples containing xanthine (5 mM) and xanthine oxidase (0.5 U mL −1 ) in 10 mM PBS and incubated for 10 min at 37 °C. Different Cu 5.4 O USNPs solutions (0, 20, 100, 1000 ng mL −1 ) were added and then the EPR signals were recorded immediately. GPx-like activity of Cu 5.4 O USNPs The GPx-like activity of Cu 5.4 O USNPs was estimated using a GPx assay kit (Solarbio, Shanghai, China) according to the manufacturer’s instructions. Glutathione (GSH) can react with 5,5′-Dithiobis-2-nitrobenzoic acid (DTNB) to form a compound with characteristic absorption at 412 nm, which could be monitored using a UV-Vis spectroscopy. During the test, GSH was oxidized to oxidized glutathione (GSSG). The decrease of GSH concentration is proportional to the catalytic activity of Cu 5.4 O USNPs. O 2 generation from H 2 O 2 catalyzed by Cu 5.4 O USNPs and CAT A commercial O 2 probe (Oxford-optronix, Oxford, UK) was utilized to measure the real-time O 2 level according to the manual instructions. Ten milliliters of PBS was poured into a small three-necked flask and stirred at 37 °C. The flask was then sealed with parafilm and rubber stoppers, and inserted with two needles for gassing. 95% N 2 /5% CO 2 gas mixture was bubbled into the flask for 20 min to create hypoxic condition. Cu 5.4 O USNPs (500 μL, 200 ng mL −1 ) and CAT (500 μL, 20 U mL −1 ) solutions were injected to the mixture, while PBS was used in the control group. Then H 2 O 2 (500 μL, 2 mM) was injected and the amount of generated O 2 was monitored at predetermined time intervals. Cell culture The human embryonic kidney 293 (HEK293) cell line was purchased from the American Type Culture Collection (ATCC). The HEK293 cells were cultured in Dulbecco’s modified Eagle’s medium (DMEM) supplemented with 10% fetal bovine serum (FBS), 100 μg mL −1 streptomycin, and 100 U mL −1 penicillin at 37 °C in an incubator supplied with a humidified atmosphere of 5% CO 2 . In vitro ROS scavenging using Cu 5.4 O USNPs To investigate the ROS scavenging ability of Cu 5.4 O USNPs in cells, HEK293 cells were seeded into 96-, 48-, and 24-well plates at the density of 1 × 10 4 cells per well, 5 × 10 4 cells per well, and 10 × 10 4 cells per well, respectively. After 24 h incubation, Cu 5.4 O USNPs with different concentrations (0–50 ng mL −1 ) were added to each group of wells and incubated for 30 min. Then, cells were treated with 250 μM H 2 O 2 and further incubated at 37 °C for 24 h. Cells seeded in 96-well plates were incubated with cell counting kit-8 (CCK-8, Dojindo, Japan) to detect the cell viability. Wells without the addition of H 2 O 2 were regarded as the negative control. Furthermore, cells seeded in 48-well plates were stained with Annexin V-FITC apoptosis detection kit (C1062, Beyotime, China) to detect the ratio of apoptotic and necrotic cells [66] . In brief, HEK293 cells in a well were collected, washed with cold PBS, and re-suspended in 195 μL binding buffer after the aforementioned incubation with H 2 O 2 for 24 h. Then, 5 μL Annexin V-FITC and 10 μL PI were sequentially added to the cell suspension and incubated at room temperature in dark for 15 min. After that, cells were analyzed by the Attune Acoustic Focusing Cytometer (Life Technologies, USA). At least 50,000 cells were analyzed in each sample. 2′,7′-Dichlorofluorescin diacetate (DCFH-DA, D6883, Sigma-Aldrich, USA), an oxidation sensitive fluorescent dye, was used to detect the intracellular ROS level according to the literature [25] . Briefly, DCFH-DA is a non-fluorescent chemical compound which could diffuse through cell membrane freely and could be hydrolyzed by intracellular esterase to DCFH. The non-fluorescent DCFH could be oxidized by the intracellular ROS to fluorescent DCF. Therefore, the quantity of intracellular ROS is correlated with the fluorescent intensity of DCF. After the aforementioned incubation with H 2 O 2 for 24 h, cells were gently rinsed thrice with serum-free medium to remove the free Cu 5.4 O USNPs. Then, a final concentration of 10 μM of DCFH-DA in serum-free medium was added to the cells and incubated in dark at 37 °C for 30 min. Afterwards, the cells were washed with serum-free medium thrice to remove unloaded DCFH-DA probe, then were imaged using a laser confocal microscope (Zeiss LSM780, Germany), and were subjected to a flow cytometry analysis to quantify the intracellular ROS levels respectively. To determine the location of Cu 5.4 O USNPs in the cells, HEK293 cells (1 × 10 6 cells) were collected after incubation with 50 ng mL −1 of Cu 5.4 O USNPs at 37 °C for 24 h. The collected cells were fixed with 2.5% glutaraldehyde at 4 °C for 2 h, then post-fixed with 1% osmium tetroxide and prepared for TEM observation. In vitro biocompatibility evaluation of Cu 5.4 O USNPs The cytotoxicity of Cu 5.4 O USNPs was determined by the CCK-8 assay in vitro. Briefly, HEK293 cells were seeded into 96-well culture plates at the density of 1 × 10 4 cells per well and incubated at 37 °C in an incubator with 5% CO 2 for 24 h. Afterwards, the cell culture medium was aspirated and fresh culture media containing various concentrations of Cu 5.4 O USNPs (0–200 ng mL −1 ) were added. After 24 or 48 h incubation, cells were gently washed once with sterile PBS and then treated with 100 μL fresh culture medium and 10 μL CCK-8 solution, and further incubated at 37 °C for 2 h. The cell viability was then quantified by measuring the absorbance value at 450 nm by a microplate reader (Thermo Varioskan Flash, USA). The hemolysis assay was performed on the basis of previously reported methods with some modifications [67] . All the animal experiments were carried out under the approval of the Institutional Animal Care and Use Committee of the Third Military Medical University (Army Medical University). Fresh whole-blood samples were collected from the orbital venous of healthy Sprague-Dawley rats. The collected blood samples were centrifugated for 15 min at 231 × g to collect erythrocytes and gently washed thrice with saline solution. Then, 3.67 mL of saline solution was added to erythrocytes collected from 1 mL blood. Afterwards, 100 μL of diluted erythrocytes suspension was mixed with 1 mL Cu 5.4 O USNP dispersion at various concentrations (50–5000 ng mL −1 ). The mixed dispersions were incubated for 3 h at 37 °C and then centrifugated for 15 min at 13800 × g before observing and recording the hemolysis phenomenon. The hemolysis ratio was quantified by measuring the absorbance value of supernatant at 540 nm with a microplate reader. Deionized water and saline solution were used as the positive and negative control, respectively. In vivo biocompatibility evaluation of Cu 5.4 O USNPs To evaluate the biocompatibility of Cu 5.4 O USNPs in vivo, BALB/c mice (aged 8–10 weeks, 20–25 g) were intravenously administrated with Cu 5.4 O USNPs at a single dose of 4 μg kg −1 . The mice injected with PBS were used as the control group. One day post injection, the blood samples were collected for complete blood panel analysis and serum biochemistry test. The serum biochemistry test included two important indicators of hepatic function as aspartate aminotransferase (AST) and alanine aminotransferase (ALT), and two indicators of kidney function as blood urea nitrogen (BUN) and creatinine (CRE). Serum IL-6 and TNF-α levels were quantified by the ELISA assay. One day and thirty days post injection, the mice were sacrificed to harvest major organs (including heart, liver, spleen, lung, and kidney) for hematoxylin and eosin (H&E) staining and histological analysis. To evaluate the in vivo toxicity of Cu 5.4 O USNPs after repeated administration, BALB/c mice (aged 8–10 weeks, 20–25 g) were intravenously administrated with Cu 5.4 O USNPs at a dose of 4 μg kg −1 every day for seven consecutive days. On eighth day, mice were sacrificed to harvest major organs for H&E staining and collect blood samples for complete blood panel analysis and serum biochemistry test. To detect the accumulation of Cu 5.4 O USNPs in the major organs after repeated administrations, BALB/c mice (aged 8–10 weeks, 20–25 g, n = 8) were intravenously administrated with Cu 5.4 O USNPs at a dose of 4 μg kg −1 every day for seven consecutive days. On the eighth day, mice were sacrificed to harvest major organs. The organs of four mice were weighed, homogenized, and then dissolved in aqua regia to calculate the percentage of injected dose per gram of tissue (%ID g −1 ) by ICP-AES. The organs of the other four mice were fixed with the mixture of 2.5% glutaraldehyde and 4% formaldehyde for 24 h, and then post-fixed with 1% osmium tetroxide and prepared for TEM observation. AKI models in mice The glycerol-induced AKI model was established according to the previously reported protocol [10] . Briefly, female BALB/c mice (aged 8–10 weeks, 20–25 g) were deprived of water but given free access to food for 15 h. After water deprivation, the two hindlimbs of mice were equally intramuscularly injected with 50% glycerol at a dose of 8 mL kg −1 . After that, all the mice had free access to water and food. Symptoms of AKI, such as a lack of activities and decreased urine output, could be observed in a few hours after glycerol injection. The cisplatin-induced AKI model was also established according to previously reported method [68] . In brief, female BALB/c mice (aged 8–10 weeks, 20–25 g) were given one time intraperitoneal injection of cisplatin (BP809, Sigma-Aldrich, USA) at a dose of 20 mg kg −1 . Mice in the treatment group were intravenously injected with Cu 5.4 O USNPs at 2 μg kg −1 dose 2 h after intraperitoneal cisplatin injection. Mice received saline injection was used as control. Three days post injection, mice were sacrificed to collect blood and renal tissues for kidney function analysis and histological analysis, respectively. Pharmacokinetics and biodistribution of Cu 5.4 O USNPs To evaluate the blood circulation half-life of Cu 5.4 O USNPs, BALB/c mice ( n = 3) with established glycerol-induced AKI model were intravenously injected with Cu 5.4 O USNPs at a dose of 2 μg kg −1 . At different time points post injection (10 min, 1, 2, 4, 8, 24, 48, and 72 h), 10 μL of whole-blood samples were collected from the mouse tail vein. The collected blood samples were dissolved in aqua regia and the concentrations of NPs were quantified by ICP-AES. A two-compartment pharmacokinetic model was utilized to calculate the pharmacokinetics parameters of Cu 5.4 O USNPs. Simultaneously, the urine and feces of mice were collected at different time points and dissolved in aqua regia to quantify the content of Cu by ICP-AES. Furthermore, the collected urine was also diluted with PBS and dropped on a carbon-coated copper grid to detect the presence of Cu 5.4 O USNPs in the urine under TEM (JEOL JEM-1400, Japan). To detect the biodistribution of Cu 5.4 O USNPs in the major organs, BALB/c mice ( n = 3) with established glycerol-induced AKI model were intravenously injected with Cu 5.4 O USNPs at a dose of 2 μg kg −1 . One day after injection, mice were sacrificed to harvest major organs including heart, liver, spleen, lung, and kidney. The tissues were weighed, homogenized, and then dissolved in aqua regia to calculate the percentage of injected dose per gram of tissue (%ID g −1 ) by ICP-AES. To study the accumulation of Cu 5.4 O USNPs in the kidney at different time periods, healthy female BALB/c mice or the ones with established AKI model ( n = 3) were intravenously injected with Cu 5.4 O USNPs at a dose of 2 μg kg −1 . At desired time points (6, 12, 24 h), three mice in each group were sacrificed. Kidney tissues were harvested, weighed, homogenized, and dissolved in aqua regia to calculate the %ID g −1 of Cu by ICP-AES. The same experiment setup was applied for another batch of mice to investigate the biodistribution of Cu 5.4 O USNPs in the GBM. At different time points (2, 24, 72 h), three mice in each group were sacrificed and a small piece of kidney tissues was fixed with the mixture of 2.5% glutaraldehyde and 4% formaldehyde for 24 h, then post-fixed with 1% osmium tetroxide and prepared for TEM observation. In vivo therapeutic outcome of Cu 5.4 O USNPs on AKI mice BALB/c mice with established AKI model were randomly divided into five groups ( n = 4): received PBS injection (control group), NAC (8 mg kg −1 ), NAC (40 mg kg −1 ), NAC (160 mg kg −1 ), and received with Cu 5.4 O USNPs at a dosage of 2 μg kg −1 , respectively. The drug or NPs were administrated once. The body weight variations in each group after treatment were monitored for 24 h. After 24 h post injection, mice were sacrificed to collect blood samples for detecting the BUN and CRE levels. The left kidneys were harvested and homogenized for the detection of renal biomarkers. The level of SOD in the kidney was detected with a SOD assay kit (19160; Sigma-Aldrich, USA). The expression levels of two important kidney injury biomarkers, heme oxygenase-1 (HO-1) and kidney injury molecule-1 (KIM-1), were detected with HO-1 (ab204524, Abcam, USA) and KIM-1 (ab213477, Abcam, USA) ELISA kits, respectively. The right kidneys were cut into two equal sections. One section was fixed with 4% paraformaldehyde and embedded in paraffin for H&E staining. The other section was frozen and embedded in optimum cutting temperature (O.C.T.) specimen matrix (Sakura, Leiden, The Netherlands) for cryostat sectioning at −20 °C. The renal tissue was sectioned into approximately 5 μm thickness. Frozen renal tissue sections were stained with DAPI (C1005, Beyotime, China) and dihydroethidium (DHE, D7008, Sigma-Aldrich, USA) at 37 °C for 30 min, gently washed thrice with PBS to remove excessive dyes and then imaged under a fluorescence microscope to qualitatively detect the ROS levels in the renal tissues. The same experiment setup was applied for another batch of mice ( n = 10) to draw the survival curves of AKI mice within 2 weeks. For therapeutic mechanism investigation of Cu 5.4 O USNPs, after 24 h post treatment, another batch of mice ( n = 3) were sacrificed to collect serum and kidney tissues for measurement of inflammatory factors by ELISA kit. In vivo therapeutic effect of Cu 5.4 O USNPs on AILI mice The acetaminophen (APAP)-induced acute liver injury model was established according to the previously reported protocol [69] . Briefly, female C57BL/6 mice (aged 8–10 weeks, 18–20 g) were deprived of food but given free access to water for 15 h. Then, 10 mice were intraperitoneally injected with APAP (dissolved in warm saline, 15 mg mL −1 ) at a dose of 300 mg kg −1 and randomly divided into two groups ( n = 5). Mice ( n = 5) without APAP injection served as control. Afterwards, all the mice had free access to water and food. Mice in the treatment group were intravenously injected with Cu 5.4 O USNPs at 6 μg kg −1 dose 2 h after APAP injection. At 24 h post injection, mice were sacrificed to collect blood and liver tissues for liver function test and histological analysis, respectively. In vivo therapeutic effect of Cu 5.4 O USNPs on wound healing To investigate the effect of Cu 5.4 O USNPs on diabetic wound healing, the STZ-induced diabetic mice model was established according to the previous literature [70] . Briefly, male BALB/c mouse (aged 8–10 weeks, 20–25 g, n = 3) were intraperitoneal injected with 100 mg kg −1 streptozotocin (STZ, Sigma-Aldrich, USA) for six consecutive days. Then all mouse were provided with normal food and water. The glucose level of mice was then monitored everyday from the tail venous blood using a blood glucose meter (Roche Diagnostics, Shanghai, China). Mice with sustained blood glucose levels exceeding 250 mg dL −1 were considered diabetic mice. These diabetic mice were used for further wounding model at 2 weeks after the initiation of STZ treatment. Full-thickness wounds were simultaneously created in the dorsal skin using a sterile 6-mm diameter punch. A green round marker (6-mm diameter) was placed beside each wound to represent the initial wound area and the wounds were photographed immediately using a digital camera. Afterwards, each wound in the treatment group was topically administrated with 20 μL of Cu 5.4 O USNPs at 400 ng mL −1 . Wounds in the control group were treated with 20 μL of PBS instead. Then, the wounds were covered with a piece of biological membrane (NPWT-1, Negative Pressure Wound Therapy Kit, China). The wounds were photographed and Cu 5.4 O was topically administrated at days 1, 4, 7, 9, 15 post-surgery, respectively. Wound areas were measured using ImageJ software. The wound healing rate was calculated based on the following formula: 
    Wound healing rate% = ( I - R)/I × 100%,
 (3) where I represented the initial wound area and R represented the remaining wound area on the determined day post-surgery. At day 15 post-surgery, mice were sacrificed to harvest wound tissues for histological analysis. The wound tissues were fixed with 4% paraformaldehyde and embedded in paraffin for H&E staining. The length of regenerated epidermis and the thickness of granulation tissues were quantified using ImageJ software. Transcriptome analysis of AKI mice BALB/c mice with established AKI model were randomly divided into two groups: received PBS injection (control group, n = 5) and received with Cu 5.4 O USNPs at a dosage of 2 μg kg −1 (experimental group, n = 5), respectively. After 24 h post injection, mice were sacrificed to collect the kidneys. Total RNA of kidney tissues were prepared using Trizol Reagent (Invitrogen, USA) according to the manufacturer’s instructions and genomic DNA was removed using DNase I (TaKara, Japan). Then RNA quality was determined by 2100 Bioanalyser (Agilent) and quantified using the ND-2000 (NanoDrop Technologies). Only high-quality RNA sample (OD 260/280 = 1.8–2.2, OD 260/230 ≥ 2.0, RIN ≥ 6.5, 28S:18S ≥ 1.0, >2 μg) was used to construct sequencing library. The RNA purification, reverse transcription, library construction, and sequencing were performed at Majorbio Bio-pharm Biotechnology Co., Ltd (Shanghai, China) using Illumina HiSeq X10 (Illumina, San Diego, CA) according to the manufacturer’s instructions. The raw paired end reads were trimmed and quality controlled by SeqPrep ( https://github.com/jstjohn/SeqPrep ) and Sickle ( https://github.com/najoshi/sickle ) with default parameters. Then clean reads were separately aligned to reference genome with orientation mode using TopHat ( http://tophat.cbcb.umd.edu/ , version2.1.1) software. For bioinformatics analysis, the expression level of each transcript was calculated according to the fragments per kilobase of exon per million mapped reads (FPKM) method. RSEM ( http://deweylab.biostat.wisc.edu/rsem/ ) was used to quantify gene abundances. DEGs were identified using R statistical package software DESeq2 ( http://bioconductor.org/packages/stats/bioc/DESeq2.html ) (fold change ≥2 and P value <0.05) with a false discovery rate (FDR) cutoff <0.05. KEGG functional enrichment analysis was performed to identify which DEGs were significantly enriched in KEGG signaling pathways at Bonferroni-corrected P value <0.05 compared with the whole-transcriptome background. KEGG enrichment analysis was performed by KOBAS 2.1.1 ( http://kobas.cbi.pku.edu.cn/download.php ). Besides, protein−protein interactions of genes were analyzed by Search Tool for the Retrieval of Interacting Genes/Proteins (STRING) algorithm ( http://www.string-db.org/ ). Quantitative real-time PCR and Western blot analysis The total RNA from kidney tissue was extracted using Trizol Reagent. cDNA was synthesized using a reverse transcription system kit according to the manufacturer’s instructions (PrimeScript™ RT reagent Kit with gDNA Eraser, RR047A, TaKaRa, Japan). Real-time PCR was performed using the TB Green Premix Ex Taq™ II kit (RR820A, Takara, Japan) following the manufacturer’s protocol. Gene expression levels were normalized to GAPDH and analyzed using the comparative cycle threshold ( F = 2 −ΔΔCt ) method. 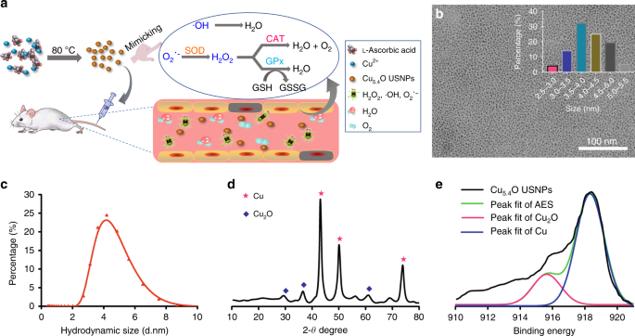Fig. 2: Preparation and characterization of Cu5.4O USNPs. aSchematic preparation of Cu5.4O USNPs.bTEM image of Cu5.4O USNPs. Inset is the statistical chart of particle size distribution. The cross-sectional area of each particle was measured by using ImageJ Software from the TEM images, with at least 500 particles counted per sample.cHydrodynamic diameter distribution of the Cu5.4O USNPs.dX-ray diffraction (XRD) pattern of the Cu5.4O USNPs, the rhombus, and star symbols represent the characteristic peaks of Cu2O and Cu, respectively.eXAES spectra of the Cu5.4O USNPs. Source data are provided as a Source Data file. Primer sequences for qRT-PCR are listed in Supplementary Table 2 . The total proteins from kidney tissue were extracted using ice-cold RIPA lysis buffer containing phosphatase and protease inhibitor cocktail (KeyGEN, China). 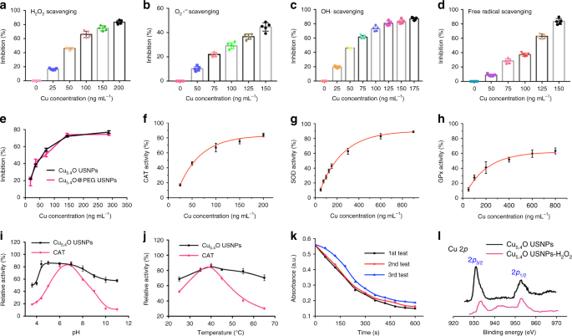Fig. 3: ROS scavenging and multienzyme-like antioxidative activity of Cu5.4O USNPs. aH2O2,bO2−,cOH·, anddfree radical scavenging ability of Cu5.4O USNPs.eH2O2-scavenging capacities of Cu5.4O USNPs and Cu5.4O@PEG USNPs.fCAT-like,gSOD-like, andhGPx-like activity of Cu5.4O USNPs.i,jThe CAT-like activity of the Cu5.4O USNPs after different treatments. H2O2(2 mM) elimination efficiencies of Cu5.4O USNPs (250 ng mL−1) and natural CAT (40 U mL−1), respectively, pretreated with differentitemperature andjpH conditions.kStability test of Cu5.4O USNPs (250 ng mL−1) when used as CAT-like catalyst at different cycles. The concentration of H2O2is 2 mM.lXPS analysis of Cu5.4O USNPs before and after treatment with H2O2. Ina–j, data represent means ± s.d. from five (a–d) or three(e–j) independent replicates. Source data are provided as a Source Data file. The concentrations of extracted proteins were determined using a BCA protein assay kit (Thermo Scientific, USA). An equal amount of protein from each sample was run in 8% SDS-PAGE gel, then transferred to polyvinylidenedifluoride (PVDF) membranes (Millipore, USA). 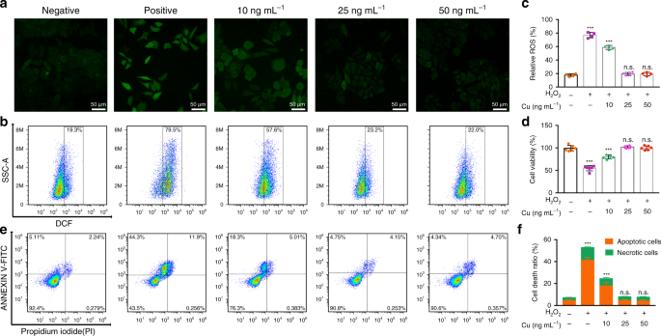Fig. 4: Scavenging ROS with Cu5.4O USNPs in vitro. aRepresentative ROS staining (green fluorescence) of HEK293 cells under different treatment conditions.bROS levels in untreated and Cu5.4O USNPs-treated HEK293 cells incubated with 250 μM H2O2.cStatistical analysis of ROS levels in HEK293 cells under different treatment conditions.dIn vitro cell viabilities of HEK293 cells under different treatment conditions.eFACS results of cell apoptosis and necrosis distribution in untreated and Cu5.4O USNPs-treated HEK293 cells.fStatistical analysis of necrotic and apoptotic cell ratios in HEK293 cells under different treatment conditions. Inc,dandf, data represent means ± s.d. from four (c,f) or six (d) independent replicates. ***P< 0.001; n.s., no significance, one-way ANOVA. Source data are provided as a Source Data file. PVDF membranes were blocked with 5% skim milk at room temperature for 2 h and then incubated with primary antibodies at 4 °C overnight, followed by incubation with secondary horseradish peroxidase-conjugated antibodies (1:1000, Sungene Biotech, China) for 1 h at room temperature. 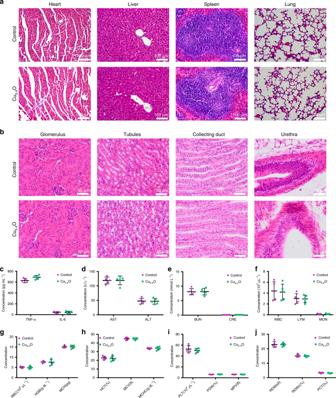Fig. 5: In vivo biocompatibility assessment of Cu5.4O USNPs. aEvaluation of in vivo toxicity of Cu5.4O USNPs to major organs (heart, liver, spleen, and lung) at 24 h after intravenous administration.bAssessment of in vivo toxicity of Cu5.4O USNPs to the kidney at 24 h after intravenous administration.cSerum levels of inflammatory factors of interleukin-6 (IL-6) and tumor necrosis factor alpha (TNF-α).dSerum levels of liver function indicators: aspartate transaminase (AST) and alanine transaminase (ALT).eSerum levels of kidney function indicators: blood urea nitrogen (BUN) and creatinine (CRE).f–jBlood parameters in normal mice (control group), and mice intravenously injected with Cu5.4O USNPs, 24 h after injection. Inc–j, data represent means ± s.d. from five independent replicates. Source data are provided as a Source Data file. The intensity of bands was visualized and determined using a ChemiDoc™ XRS detection system (Bio-Rad, USA). Primary antibodies used were: NF-κB p65 (L8F6), phospho-NF-κB p65 (Ser536, E1Z1T), IκB-α (L35A5), phospho-IκB-α (Ser32/36, 5A5) (1:1000, Cell Signaling Technology, USA) and β-actin (1:1000, Sungene Biotech, China). 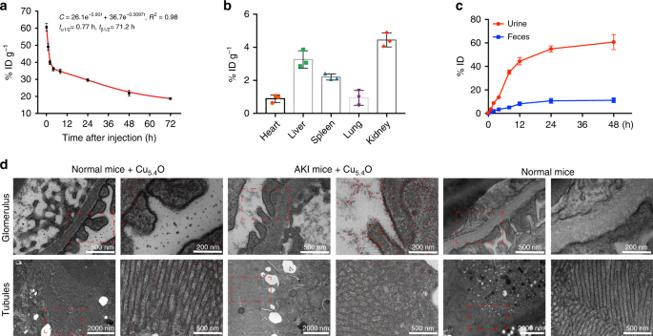Fig. 6: Pharmacokinetics, biodistribution, and clearance of Cu5.4O USNPs in AKI mice. aIn vivo blood pharmacokinetic curves after intravenous injection of Cu5.4O USNPs.bBiodistribution of Cu5.4O USNPs in major organs at 24 h post injection.cCumulative urine and feces excretion at different time points.dBiodistribution of Cu5.4O USNPs in renal tissues by TEM observation. Red dashed lines indicate the magnified area. Dots with red pseudocolor indicate Cu5.4O USNPs. Ina–c, data represent means ± s.d. from three independent replicates. Source data are provided as a Source Data file. 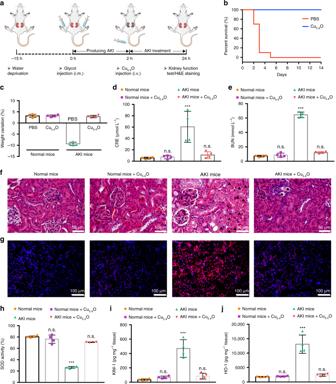Fig. 7: Ttherapeutic efficiency of Cu5.4O USNPs on AKI mice. aSchematic illustration of the establishment and treatment schedule of AKI mice.bSurvival curves of AKI mice with different treatment.cWeight variation of AKI mice at 24 h after treatment with Cu5.4O USNPs. Serum levels ofdCRE andeBUN in AKI mice at 24 h after different treatment.fH&E staining of kidney tissues from each group. Triangles indicate the formation of casts.gDihydroethidium (red fluorescence) and DAPI (blue fluorescence) staining of kidney tissues from each group.hSOD,iKIM-1, andjHO-1 levels measured in renal tissue homogenates from each group. Inc–eandh–j, data represent means ± s.d. from four independent replicates (***P< 0.001; n.s., no significance, One-way ANOVA). Source data are provided as a Source Data file. The primary images (Fig. S31 ) were cropped for presentation. 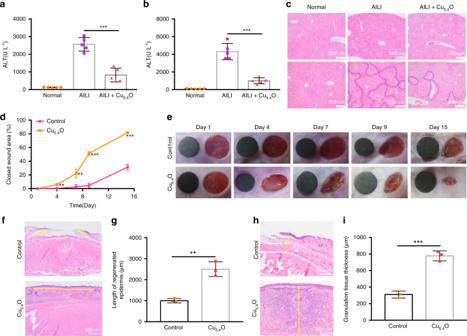Fig. 8: Therapeutic efficiency of Cu5.4O USNPs on AILI and wound healing. Serum levels ofaAST andbALT in AILI mice at 24 h after different treatment.cH&E staining of liver tissues from each group. Blue dashed lines indicate the range of hepatic necrosis. The percentage ofdclosed diabetic wound area and representative macroscopic appearance ofediabetic wound at different time points. A 6-mm-diameter standard green disc was used as the reference when taking photos.fRepresentative histological images andgquantitative determination of the length of regenerated epidermis on day 15 post-surgery. The yellow double-headed arrows indicate the regenerated epidermis.hRepresentative histological images andiquantitative measurement of granulation tissue thickness on day 15 post-surgery. The yellow double-headed arrows indicate the granulation tissue. Ina,b, data represent means ± s.d. from five independent replicates (one-way ANOVA). Ind,gandi, data represent means ± s.d. from three independent replicates (Student’st-test, **P< 0.01; ***P< 0.001). Source data are provided as a Source Data file. 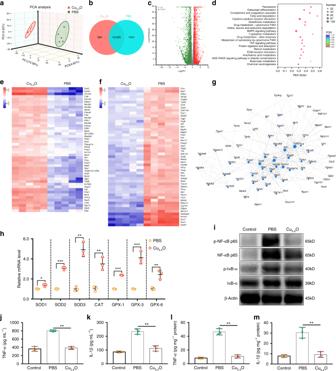Fig. 9: Therapeutic mechanisms of Cu5.4O USNPs on AKI. aPrincipal component analysis (PCA) was performed based on differentially expressed genes from the kidneys of two groups. Each data point corresponds to the PCA analysis of each sample.bVenn diagram of the transcriptomic profiles between Cu5.4O USNPs and PBS groups.cVolcano plots showing the identified upregulated and downregulated genes by Cu5.4O USNPs.dKEGG pathway enrichment analysis of the identified differentially expressed genes. The 20 most significantly enriched pathways are shown. Heat maps of significantlyeupregulated andfdownregulated genes involved in the oxidative stress after Cu5.4O USNPs treatment (fold change ≥2 andP< 0.05).gProtein–protein interaction network of differentially expressed genes involved in the oxidative stress.hqRT-PCR analysis of the mRNA expression levels of antioxidant genes.iWestern blot analysis of the expression of phospho-NF-κB p65, total NF-κB p65, phospho-IκB-α, and total IκB-α in kidney tissues of AKI mice. Serum levels ofjTNF-α andkIL-1β. Renal levels oflTNF-α andmIL-1β. Inh,j–m, data represent means ± s.d. from three independent replicates, andPvalues were calculated by Student’st-test (h) and one-way ANOVA (j–m). *P< 0.05; **P< 0.01; ***P< 0.001. Source data are provided as a Source Data file. Reporting summary Further information on research design is available in the Nature Research Reporting Summary linked to this Article.